A doublecortin containing microtubule-associated protein is implicated in mechanotransduction inDrosophilasensory cilia Mechanoreceptors are sensory cells that transduce mechanical stimuli into electrical signals and mediate the perception of sound, touch and acceleration. Ciliated mechanoreceptors possess an elaborate microtubule cytoskeleton that facilitates the coupling of external forces to the transduction apparatus. In a screen for genes preferentially expressed in Drosophila campaniform mechanoreceptors, we identified DCX-EMAP, a unique member of the EMAP family (echinoderm–microtubule-associated proteins) that contains two doublecortin domains. DCX-EMAP localizes to the tubular body in campaniform receptors and to the ciliary dilation in chordotonal mechanoreceptors in Johnston's organ, the fly's auditory organ. Adult flies carrying a piggyBac insertion in the DCX-EMAP gene are uncoordinated and deaf and display loss of mechanosensory transduction and amplification. Electron microscopy of mutant sensilla reveals loss of electron-dense materials within the microtubule cytoskeleton in the tubular body and ciliary dilation. Our results establish a catalogue of candidate genes for Drosophila mechanosensation and show that one candidate, DCX-EMAP, is likely to be required for mechanosensory transduction and amplification. Mechanotransduction is the process by which a mechanical force impinging on a cell produces an intracellular signal. This signal may function locally within the tissue to regulate cellular motility, growth or differentiation [1] or it may be transmitted to the central nervous system where it can lead to the perception of sound, touch or accelerations [2] . Mechanosensory cells often contain elaborate cytoskeletal structures that provide a mechanical link from the external stimulus to the receptor module. A well-studied example of such a cytoskeletal linkage apparatus is the hair bundle of hair cells, the receptor cells underlying the senses of hearing and balance in the vertebrate inner ear. Shearing of adjacent actin-filled stereocilia within the bundle tenses extracellular links and leads to the opening of transduction channels located close to the apical tips of the stereocilia [3] . In addition to actin-based mechanoreceptors such as hair cells, vertebrates and invertebrates contain microtubule-based sensory cells. Ciliated and non-ciliated sensory neurons in Caenorhabditis elegans ( C. elegans ) mediate the response to touch [4] . Ciliated epithelial cells in the kidney detect fluid flow [5] , and ciliated receptor neurons in insect bristle receptors, campaniform sensilla and chordotonal organs sense forces associated with touch, air flow, cuticle deformation, gravity and sound [6] . The transduction apparatus of auditory chordotonal receptor neurons in the Drosophila antenna has been shown to be functionally equivalent to that of hair cells in that it can be described by serially arranged force-gated transduction channels, adaptation motors and gating springs [7] . Correlates of auditory transducer gating and associated amplification have been identified in the fly's antennal mechanics, but proteins that are required for transducer function have not been identified as yet. In this study, we used DNA microarrays to identify genes that are specifically expressed in Drosophila campaniform receptors. Our reasoning was that such genes may include novel mechanotransduction genes that have not been found in behavioural screens [8] , [9] . We identified a unique doublecortin-domain-containing echinoderm–microtubule-associated protein (DCX-EMAP, CG42247) as a candidate for a mechanoreceptor-specific protein in flies. EMAP was first identified in sea urchins ( Strongylocentrotus purpuratus ) [10] . All EMAP family members share a common conserved HELP domain (HELP; hydrophobic echinoderm–microtubule-associated-like protein) located at an acidic N-terminus and multiple C-terminal WD-40 domains [11] . Some EMAP homologues have a role in cell division [12] , [13] , [14] , [15] , [16] , and others are expressed in neurons [17] , including the C. elegans homologue, which is expressed in muscles and mechanosensory cells [18] . In contrast to EMAP homologues from other organisms, DCX-EMAP lacks the coiled-coil domain, but possesses two doublecortin (DCX) domains at its N-terminus. Doublecortin, mutations in the gene of which leads to X-linked lissencephaly in humans, is a microtubule-associated protein found in migrating neurons [19] , [20] . Doublecortin is a microtubule-stabilizing protein that suppresses catastrophes (the conversion of a growing microtubule to a shrinking one), stimulates microtubule nucleation and promotes the formation of 13-protofilament microtubules [21] , [22] . In this paper, we show that DCX-EMAP is necessary for auditory transducer gating and amplification in Drosophila chordotonal receptor cells, as well as for the formation of microtubule-associated electron-dense material within the sensory dendrites of campaniform and chordotonal neurons. Our findings identify DCX-EMAP as the first invertebrate protein that is essential for auditory transducer function, and supports previous suggestions that the tubular body of campaniform receptors and the ciliary dilation of chordotonal receptors may be sites of mechanosensory transduction [23] , [24] . Screen for candidate mechanostransduction genes We used DNA microarrays (Affymetrix) to identify genes of which the expression is increased in campaniform mechanosensilla of the fly's halteres. Halteres are vestigial hindwings that function as gyroscopes [25] . They are composed of three segments: the large distal segment, the capitellum, functions as an inertial mass; and the proximal segments, the pedicel and scabellum, contain arrays of campaniform sensilla that detect cuticular stresses generated when the fly accelerates and the capitellum moves relative to the body ( Supplementary Fig S1 ). The proximal segments contain 186 campaniform sensilla, whereas only 18 bristle receptors are housed by the capitellum [26] . Because, the capitellum is ∼ 10 times larger in volume than the pedicel and scabellum combined, the proximal segments are ∼ 100-fold enriched in mechanosensory cells over the capitellum. The other cell types are primarily epithelial cells. We therefore expected that tissue from the proximal segments would be ∼ 100-fold enriched in RNA expressed specifically in mechanosensilla (compared with the capitellum), but both tissues would have approximately the same expression levels of epithelial genes. Because each mechanosensillum contains a mechanoreceptor cell and supporting cells, we reasoned that messages specifically expressed in mechanoreceptors, including possible mechanotransduction genes, would be enriched in the proximal-segment tissue. To compare the relative expression of genes in mechanoreceptor-rich and mechanoreceptor-poor tissues, we extracted RNA separately from the two proximal segments and the one distal segment of 50 halteres. RNA was also extracted from the thoracic ganglion to serve as a neuronal model tissue. Because the yield was low, RNA was amplified before hybridization with DNA microarrays containing multiple 25-mer oligonucleotide probes for ∼ 13,000 different Drosophila genes. After scanning and processing of arrays to remove technical variances (see Supplementary Information ), differences between tissues were calculated from a linear model fit. In particular, a log 2 -ratio M PC comparing the expression levels in the two proximal segments (hereafter called 'pedicel') with the capitellum was computed. Similarly, the log 2 -ratio M PN compares gene expression in the pedicel compared with that in the thoracic ganglion. Supplementary Data contain the top 625 genes (our candidate gene list) ranked by the probability of a difference between pedicel and capitellum. This corresponds to 4.8% of the total genes (625 out of 13,000). To determine whether our DNA microarray experiments identified genes overexpressed specifically in mechanosensory cells, we carried out several additional tests. First, we performed quantitative real-time PCR (qRT–PCR) on 12 candidate genes, comparing pedicel and capitellum tissue. There was a highly statistically significant correlation between the log 2 of the ratio of qRT–PCR values and M values ( t =4.7, P <0.0003, Supplementary Fig S2 and Supplementary Table S1 ). Second, because campaniform receptors are ciliated sensory cells, we expected to find cilia-specific genes. In accordance with this expectation, our candidate list includes 36 flagellar and basal body proteome genes defined by Li et al . [27] out of the 231 flagellar and basal body genes represented in our array. The list thus contains 16% of the flagellar and basal body genes, which is significantly more ( P <10 −9 ) than the 5% coverage of total genes. We also found 16 of the 26 ciliary compartment genes defined by Avidor-Reiss et al . [28] as required for ciliated receptor outer-segment formation or function ( Supplementary Data ). Again, these genes are significantly overrepresented in our list ( P <10 −14 ). Third, we found TRPN1 (also known as nompC ), the only candidate mechanotransduction gene to date [29] , being upregulated. 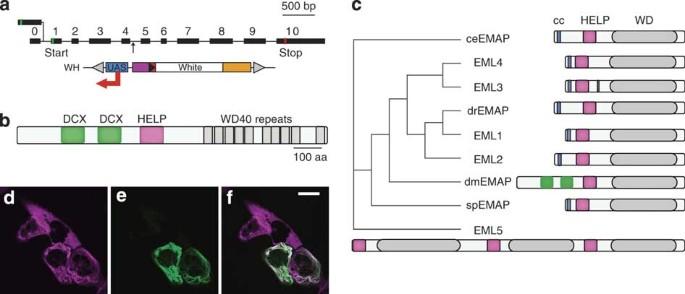Figure 1: DCX-EMAP, a doublecortin-domain-containing member of the echinoderm–microtubule-associated protein family. (a) The exon–intron structure of CG42247 showing the piggyBac (f02655) insertion into the intron between exons 4 and 5. (b) The domain structure of the DCX-EMAP protein. Two (one for the truncated form) N-terminal doublecortin domains (DCX) are followed by a HELP domain. The C terminus of the 819 aa protein consists of 10 WD40 domains, shown in grey. (c) The EMAP family tree (S. purpuratus, C. elegans, D. melanogaster, D. rerio) and the five mammalian (mouse EML 1-5) EMAP homologues are shown (similarity matrix, blosum; parameters: neighbour joining; tie breaking, systematic). (d–f) U2OS cells expressing α-tubulin-mCherry (d) transfected with DCX-EMAP-EGFP (e), and overlay (f) showing co-localization between microtubules and DCX-EMAP and large microtubule bundles not observed in non-transfected cells (scale bar, 20 μm). Finally, data mining using FlyMine and the BDGB in situ database [30] , [31] confirmed that the majority of genes in the candidate gene list are expressed in sensory cells ( Table 1 ). The BDGP in situ database contains images of patterns of gene expression during embryogenesis for Drosophila genes represented in non-redundant sets of Drosophila ESTs. All expression patterns are annotated using controlled vocabulary (ImaGO terms). Table 1 shows terms enriched in our candidate gene list and the corresponding P -value. The terms displayed in Table 1 demonstrate that genes with an expression in sensory structures are clearly enriched in our candidate gene list. In fact, we can conclude that genes expressed in sensory cells form the majority of genes in the candidate gene list ( Supplementary Data ). Table 1 Enrichment of gene expression terms in the candidate gene list ( Supplementary Data ). Full size table As possible candidates for the transduction channel, we identified two members of the transient receptor potential (TRP) family, TRPN1 ( M PC =2.2; M PN =1.4) [29] and wtrw (CG31284), recently described to be involved in hygrosensation ( M PC =4.2, M PN =3.5) [32] . Given the correlation between microarray intensity levels and RNA levels measured by qRT–PCR, and the significant overrepresentation of cilial, basal-body and genes known to be expressed in mechanoreceptors, it seems likely that our candidate gene list contains novel genes involved in mechanosensory transduction. DCX-EMAP is a candidate mechanotransduction gene One of our candidate genes is DCX-EMAP ( Fig. 1 ), which is mentioned in the Introduction section. DCX-EMAP is more than sixfold enriched in the haltere pedicel compared with the capitellum ( M PC =2.6) and neuronal control tissue ( M PN =2.7). This enrichment, which is highly significant ( B PC =5.3, B PN =6.2; corresponding to probabilities of 99.5 and 99.8%), was confirmed by qRT–PCR ( Supplementary Information ). In situ hybridization (BDGP database) shows that, in Drosophila embryos, DCX-EMAP is specifically expressed in mechanoreceptor cells [31] . DCX-EMAP displays an unusual domain architecture compared with other members of the EMAP family: it lacks the coiled-coil domain and has two DCX domains ( Fig. 1b,c ). To test for its ability to bind microtubules, DCX-EMAP was expressed in U2OS cells. DCX-EMAP co-localizes with microtubules ( Fig. 1d-f ); moreover, it bundles microtubules in these cells. Thus, the candidate gene list includes one candidate that encodes a microtubule-associated protein. Figure 1: DCX-EMAP, a doublecortin-domain-containing member of the echinoderm–microtubule-associated protein family. ( a ) The exon–intron structure of CG42247 showing the piggyBac (f02655) insertion into the intron between exons 4 and 5. ( b ) The domain structure of the DCX-EMAP protein. Two (one for the truncated form) N-terminal doublecortin domains (DCX) are followed by a HELP domain. The C terminus of the 819 aa protein consists of 10 WD40 domains, shown in grey. ( c ) The EMAP family tree ( S. purpuratus, C. elegans, D. melanogaster, D. rerio ) and the five mammalian (mouse EML 1-5) EMAP homologues are shown (similarity matrix, blosum; parameters: neighbour joining; tie breaking, systematic). ( d–f ) U2OS cells expressing α-tubulin-mCherry ( d ) transfected with DCX-EMAP-EGFP ( e ), and overlay ( f ) showing co-localization between microtubules and DCX-EMAP and large microtubule bundles not observed in non-transfected cells (scale bar, 20 μm). Full size image We decided to follow-up on the possible role of DCX-EMAP in mechanotransduction because: (1) microtubules are a prominent cytoskeletal feature of ciliated mechanoreceptors, and (2) we, along with others, have shown that, in zebrafish, drEMAP is expressed in neuromasts along the lateral line organ ( Supplementary Fig S3 ) [33] , [34] , suggesting that EMAP may be an evolutionarily conserved mechanotransduction gene. DCX-EMAP defects cause uncoordination and deafness To determine whether defects in DCX-EMAP have an effect on Drosophila behaviour, we examined a piggyBac [35] , [36] insertion line ( Fig. 1a ). The piggyBac insertion f02655 (Bloomington stock number 18573) is inserted into the intron between exons 4 and 5 of DCX-EMAP ( Fig. 1a ). Flies that are homozygous for this insertion, or that are transheterozygous for the insertion and for either of two small chromosomal deletions (Df(3L)BSC441, Df(3L)ED217), that is, they have an insertion in one copy of the chromosome and a deletion of the DCX-EMAP gene region in the other copy, showed a mild degree of uncoordination, including unstable walk, spread wing position, extensive grooming, the inability to initiate stable flight and sluggishness. We characterized flight initiation using an assay developed by Benzer: [37] homozygous as well as transheterozygous flies performed significantly worse than wild-type controls ( Fig. 2a,b ). Flies homozygous and transheterozygous for the piggyBac insertion are indistinguishable in their phenotype. Therefore, we conclude that the piggyBac insertion is a functional null. Heterozygous flies showed a slight decrease in flight initiation performance compared with wild-type flies. We do not believe that this is due to a dominant-negative effect of the piggyBac insertion because piggyBac excision flies also showed a similar small decrease in flight-initiation performance ( Fig. 2b ). Rather, we attribute the slight impairment seen in heterozygous and excision flies to the susceptibility of this complex behaviour to slight differences in genetic backgrounds. 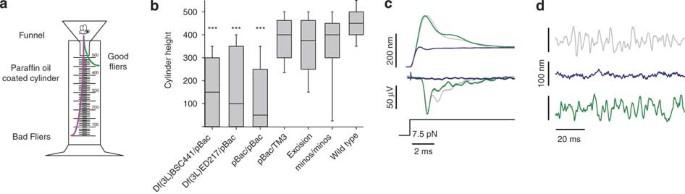Figure 2: Mutations in DCX-EMAP are associated with uncoordination and deafness in flies. (a) Flight initiation assay37. (b) Results from the flight initiation assay displayed as box plots. The box marks the 25th and 75th percentile and the median (middle line). The whiskers mark the 10th and 90th percentile. Triple asterisk,P<0.001; unpairedt-test compared with wild type;n=27 (Df(3L)BSC441/piggyBac), 41 (Df(3L)ED217/piggyBac), 51 (pBac/pBac), 46 pBac/TM3), 34 (excision), 84 (minos/minos), 118 (wild type). (c) Force step (lower trace)-evoked CAP responses (middle traces) are absent in the antennal nerves of f02655 DCX-EMAP mutants (blue), whereas robust CAP responses can be recorded from wild-type (grey) and f02655 excision controls (green). Upper panel: on step actuation, the movement of the antennal receivers of controls, but not mutants, displays the characteristic overshoot that associates with the opening of transduction channels. (d) Unstimulated fluctuations of the antennal receivers of f02655 DCX-EMAP mutants and controls. Colour code as in (c). Figure 2: Mutations in DCX-EMAP are associated with uncoordination and deafness in flies. ( a ) Flight initiation assay [37] . ( b ) Results from the flight initiation assay displayed as box plots. The box marks the 25th and 75th percentile and the median (middle line). The whiskers mark the 10th and 90th percentile. Triple asterisk, P <0.001; unpaired t -test compared with wild type; n =27 (Df(3L)BSC441/piggyBac), 41 (Df(3L)ED217/piggyBac), 51 (pBac/pBac), 46 pBac/TM3), 34 (excision), 84 (minos/minos), 118 (wild type). ( c ) Force step (lower trace)-evoked CAP responses (middle traces) are absent in the antennal nerves of f02655 DCX-EMAP mutants (blue), whereas robust CAP responses can be recorded from wild-type (grey) and f02655 excision controls (green). Upper panel: on step actuation, the movement of the antennal receivers of controls, but not mutants, displays the characteristic overshoot that associates with the opening of transduction channels. ( d ) Unstimulated fluctuations of the antennal receivers of f02655 DCX-EMAP mutants and controls. Colour code as in ( c ). Full size image Flies homozygous for insertion f02655 are severely hearing impaired. The mechanically evoked compound action potentials (CAP) recorded from the ears of wild-type flies and excision controls are absent in mutants ( Fig. 2c , middle traces). Two lines of evidence suggest that this hearing impairment is due to a defect in the gating of transduction channels. First, the large peak in the evoked displacement of the antenna that arises from compliance associated with the gating of mechanotransducer channels in Johnston's organ [38] is greatly diminished in the mutant ( Fig. 2c , upper traces). Second, the large spontaneous twitches of the arista of control flies, which are thought to reflect the active mechanical amplification arising from the feedback between mechanotransducer channels and molecular motors [7] , are strongly reduced in magnitude ( Fig. 2d ) in the receivers of DCX-EMAP mutant flies. Thus, the ears of DCX-EMAP mutants have impaired mechanical and electrical responses. To achieve a better understanding of the observed phenotypes, we conducted a more detailed analysis of the mechanics of stimulated and unstimulated receivers, as well as the corresponding nerve responses of DCX-EMAP mutants, and wild-type and piggyBac excision controls. The receivers of DCX-EMAP mutants display a reduced total fluctuation power and a shift in their best frequencies to higher values, as found in dead flies ( Fig. 3a ) [39] . The energy gain for amplification, calculated from the spectral data, is absent in DCX-EMAP mutants, but is restored to wild-type levels in piggyBac excision controls ( Fig. 3b ). To directly test for nonlinear feedback amplification, we exposed the sound receivers (aristae) of mutant and control flies to tones of different intensities. In response to pure tones of different intensities, receivers of wild-type and excision control flies display a characteristic nonlinear compression, which makes the receiver more sensitive when the sound is faint ( Fig. 3c ) [40] . In f02655 mutants, this nonlinear effect was lost. Sensitivity gains calculated from these displacement responses showed a sevenfold gain in sensitivity due to nonlinear amplification for control flies ( Fig. 3c , bottom). In contrast, the receivers of f02655 mutants constantly displayed low sensitivity over the entire range of stimulus intensities, with a mean sensitivity gain of ∼ 1, confirming that amplification is entirely lost ( Fig. 3c , bottom). 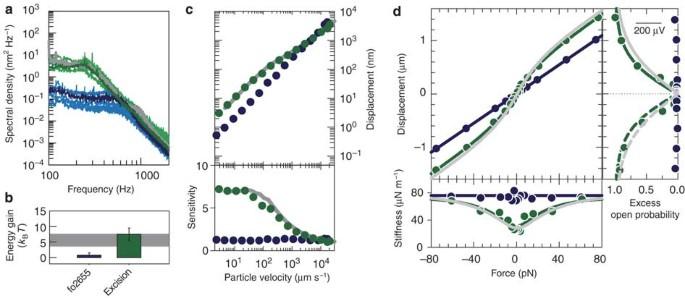Figure 3: Transduction and amplification are impaired in DCX-EMAP mutants. (a) Power spectra of unstimulated receiver vibrations in the DCX-EMAP mutant (blue traces in all panels), wild-type (grey traces) and f02655 excision controls (green). (b) Energy gain provided by active amplification deduced from the power spectra in (a)49. The range of wild-type values (one standard deviation around the mean) is marked in grey. Error bars display one standard deviation. (c) Response to pure-tone stimuli. Upper panel: Displacement response of the antennal receiver versus stimulus particle velocity. Lower panel: Mechanical sensitivity of the receiver plotted against particle velocity. Wild-type: grey, f02655 mutant: blue circles, f02655 excision control: green circles. (d) Response to force steps. Upper left panel: Displacement response of the receiver as a function of the stimulus force. Lower panel: The corresponding slope stiffness drops for small force amplitudes in wild type (grey) and excision controls, whereas it is constant for DCX-EMAP f02655 mutants (blue). The displacement-force relations of excision and control flies and the corresponding slope stiffnesses are well described by fits of a symmetric gating-spring model38. Right panel: CAP responses and predicted excess open probability versus receiver displacement. For wild type (grey) and excision controls (green), the mechanically evoked CAP response closely follows the excess open probability predicted from displacement data using a symmetric gating-spring model (solid lines for pO(×peak), dashed lines for pO(-×peak)7). Figure 3: Transduction and amplification are impaired in DCX-EMAP mutants. ( a ) Power spectra of unstimulated receiver vibrations in the DCX-EMAP mutant (blue traces in all panels), wild-type (grey traces) and f02655 excision controls (green). ( b ) Energy gain provided by active amplification deduced from the power spectra in ( a ) [49] . The range of wild-type values (one standard deviation around the mean) is marked in grey. Error bars display one standard deviation. ( c ) Response to pure-tone stimuli. Upper panel: Displacement response of the antennal receiver versus stimulus particle velocity. Lower panel: Mechanical sensitivity of the receiver plotted against particle velocity. Wild-type: grey, f02655 mutant: blue circles, f02655 excision control: green circles. ( d ) Response to force steps. Upper left panel: Displacement response of the receiver as a function of the stimulus force. Lower panel: The corresponding slope stiffness drops for small force amplitudes in wild type (grey) and excision controls, whereas it is constant for DCX-EMAP f02655 mutants (blue). The displacement-force relations of excision and control flies and the corresponding slope stiffnesses are well described by fits of a symmetric gating-spring model [38] . Right panel: CAP responses and predicted excess open probability versus receiver displacement. For wild type (grey) and excision controls (green), the mechanically evoked CAP response closely follows the excess open probability predicted from displacement data using a symmetric gating-spring model (solid lines for p O (× peak ), dashed lines for p O (-× peak ) [7] ). Full size image To test for the mechanical signatures of transducer gating, we exposed the receivers of mutant and control flies to a series of force steps while measuring their displacement responses. When deflected by a force step (lower traces in Fig. 2c ), control receivers display an initial displacement peak (upper traces in Fig. 2c ) that nonlinearly scales with the external force ( Fig. 3d ). This nonlinear gating compliance, which arises from the gating of auditory transduction channels and conforms to the gating spring model of hair cell transduction (green lines in Fig. 3d ), was lost in f02655 EMAP mutants ( Fig. 3d ). In controls, mechanically evoked CAP responses ( Fig. 3d , right panel) followed the transducer open probability that can be deduced from the receiver's nonlinear gating compliance with a symmetric version of the gating spring model (green line in Fig. 3d , right panel). In accordance with the loss of this gating compliance, CAP responses in f02655 mutants were also lost (blue circles in Fig. 3d ). Hence, DCX-EMAP mutants lack both auditory transducer gating and mechanical feedback amplification and, accordingly, fail to generate mechanically evoked electrical signals in the antennal nerve. Ultrastructural analysis of sensory dendrites To examine the structural integrity of sensory cells in DCX-EMAP mutants, we used high-pressure freezing to visualize the sensory dendrites in wild-type and mutant mechanoreceptors by electron microscopy. Wild-type tubular bodies in campaniform receptors are characterized by a dense array of parallel microtubules; in the distal part of the tubular body, this structure flattens and becomes fan shaped ( Fig. 4a ) [6] . Here, microtubules are connected by an electron-dense material ( Fig. 4b–e ). In f02655 homozygous flies, this electron-dense material was missing, and the parallel organization of microtubules in the distal tubular body was severely disturbed ( Fig. 4f–i ). Despite the ultrastructural alterations in the mutant, the general shape of the distal tubular body remained the same as in wild-type flies, and no other anatomical defects were observed. 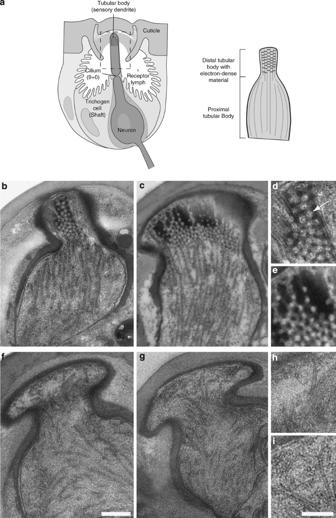Figure 4: The ultrastructure of the tubular body in f02655 campaniform receptors in theDrosophilahaltere is altered. (a) Schematic drawing of the campaniform receptor. The tubular body of the receptor is marked and illustrated separately (right panel). (b,c) Electron micrographs of the sensory dendrite in wild-type campaniform receptors in the haltere. The distal part of the tubular body shows characteristic electron-dense material. (d,e) Electron-dense material in the distal tubular body at higher magnification. (f,g) Electron micrographs of f02655 campaniform receptors. The electron-dense material in the distal tubular body is missing. Microtubules in the proximal tubular part seem disorganized. (h,i) Distal tubular bodies of f02655 campaniform receptors at higher magnification. Scale bars represent 0.5 μm (f) and 250 nm (i). Figure 4: The ultrastructure of the tubular body in f02655 campaniform receptors in the Drosophila haltere is altered. ( a ) Schematic drawing of the campaniform receptor. The tubular body of the receptor is marked and illustrated separately (right panel). ( b , c ) Electron micrographs of the sensory dendrite in wild-type campaniform receptors in the haltere. The distal part of the tubular body shows characteristic electron-dense material. ( d , e ) Electron-dense material in the distal tubular body at higher magnification. ( f , g ) Electron micrographs of f02655 campaniform receptors. The electron-dense material in the distal tubular body is missing. Microtubules in the proximal tubular part seem disorganized. ( h , i ) Distal tubular bodies of f02655 campaniform receptors at higher magnification. Scale bars represent 0.5 μm ( f ) and 250 nm ( i ). Full size image The sensory dendrites of the chordotonal receptors of Johnston's organ are characterized by a long cilium that contains a single bulge-like modification in its middle called the ciliary dilation ( Fig. 5a ) [41] . Here, the doublet microtubules of the 9+0 cilium bend around electron-dense material that displays a distinct hexagonal pattern ( Fig. 5b,c ). This electron-dense material was entirely missing in DCX-EMAP f02655 mutants ( Fig. 5d,e ). Notwithstanding this loss, the dilation was of normal shape and size: microtubules still bend within the dilation and seemed to be associated with the membrane (arrowhead, Fig. 5e ). 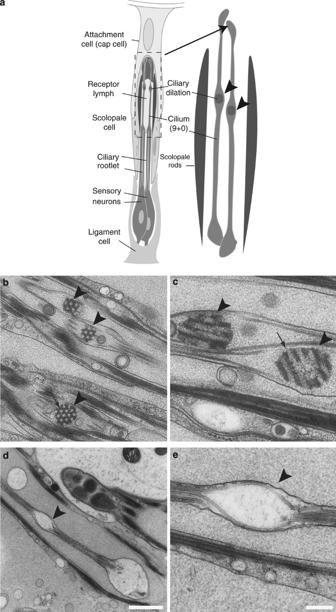Figure 5: Mutant f02655 sensory neurons of Johnston's organ display an altered ultrastructure. (a) Schematic representation of Johnston's organ in sensory neurons ofDrosophilaantenna. The region with the ciliary dilation is marked and illustrated separately (right part). (b,c) Electron micrographs of ciliary dilations (arrowheads) in wild-type chordotonal neurons with electron-dense material in the ciliary dilation (arrows point towards regular holes and channels in the electron-dense material). (d,e) Chordotonal neuron of f02655 flies with 'empty' ciliary dilations. Note how the microtubules are still bent as in wild-type dilations. Scale bars represent 1 μm (d) and 250 nm (e), arrowheads point towards ciliary dilation. Figure 5: Mutant f02655 sensory neurons of Johnston's organ display an altered ultrastructure. ( a ) Schematic representation of Johnston's organ in sensory neurons of Drosophila antenna. The region with the ciliary dilation is marked and illustrated separately (right part). ( b , c ) Electron micrographs of ciliary dilations (arrowheads) in wild-type chordotonal neurons with electron-dense material in the ciliary dilation (arrows point towards regular holes and channels in the electron-dense material). ( d , e ) Chordotonal neuron of f02655 flies with 'empty' ciliary dilations. Note how the microtubules are still bent as in wild-type dilations. Scale bars represent 1 μm ( d ) and 250 nm ( e ), arrowheads point towards ciliary dilation. Full size image The electron-dense materials in the tubular body and in the ciliary dilation both span the area between microtubules. In thin sections, the materials display regular, hexagonally spaced holes of diameter 50 nm and centre-to-centre spacing of ∼ 70 to 100 nm. These holes are almost spherical in the tubular body (arrow in Fig. 4d ) but cylindrical in the ciliary dilation (arrows in Fig. 5b,c ). When DCX-EMAP is disrupted, these electron-dense materials, but apparently no other subciliary structures, are lost. DCX-EMAP localization in sensory dendrites We determined the subcellular localization of DCX-EMAP within sensory neurons. We cloned the full-length DCX-EMAP gene and a shorter splice variant lacking the first exon, and therefore the first DCX domain, and used them to make upstream activating sequence (UAS) constructs with a C-terminal EYFP or dsRED tag. When driven with a pan-neural Gal4 driver, fluorescently tagged DCX-EMAP localized exclusively to subcompartments within the sensory dendrites of mechanoreceptor cells ( Fig. 6 ). This localization was identical for the full-length and truncated variant of DCX-EMAP, both of which labelled specific dendritic structures in campaniform and chordotonal receptor cells. In campaniform receptors ( Fig. 6a–d ), DCX-EMAP localized to the tubular body (arrowhead in Fig. 6c ). In the chordotonal receptors of Johnston's organ ( Fig. 6e–h ), DCX-EMAP localized to the ciliary dilation (arrowhead in Fig. 6g ). To confirm this finding by a second independent experiment, we coexpressed DCX-EMAP-dsRed with GFP-centrosomin (CNN-GFP), which is a centrosome/basal-body marker. As displayed in Fig. 6m–p , DCX-EMAP and CNN-GFP do not co-localize. DCX-EMAP can be found distal to the basal body/rootlet structures marked by GFP-CNN. We therefore conclude that DCX-EMAP localizes to the ciliary dilation. At the light microscopy level, fluorescently tagged DCX-EMAP thus localizes to specific ciliary subcompartments: the tubular body in campaniform receptors and the ciliary dilation in chordotonal neurons. This correlates with the sites of ultrastructural defects in DCX-EMAP mutants. 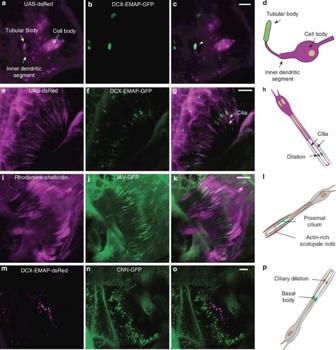Figure 6: DCX-EMAP localization in campaniform receptors. (a) UAS-dsRED localization in a wing-vein campaniform receptor. (b) UAS-EMAP-GFP localizes to the tubular body and is not detectable in other cellular compartments. (c) Merge of panelsaandb. Arrowhead points toward the tubular body. (d) Schematic of the campaniform receptor. (e) GFP-tubulin showing sensory cilia. (f) EMAP-dsRed localizes to ciliary dilations. (g) Merge of panelseandf(sensory cilia are marked by arrows). (h) Schematic of DCX-EMAP localization in chordotonal receptors. (i) Rhodamine-phalloidin staining the actin rods within scolopale cells. (j) UAS-IAV-GFP expressed in chordotonal neurons using DJ648-Gal4. (k) Merge showing that IAV-GFP localizes to the proximal part of the cilia. (l) Schematic of IAV localization. (m) UAS-DCX-EMAP-dsRed expressed in chordotonal neurons of Johnston's organ (n) UAS-CNN-GFP. (o) Merge of panels m and n showing the localization of DCX-EMAP-dsRed distal to CNN-GFP. (p) Schematic of DCX-EMAP-dsRed and CNN-GFP localization. All scale bars are 5 μm. Figure 6: DCX-EMAP localization in campaniform receptors. ( a ) UAS-dsRED localization in a wing-vein campaniform receptor. ( b ) UAS-EMAP-GFP localizes to the tubular body and is not detectable in other cellular compartments. ( c ) Merge of panels a and b . Arrowhead points toward the tubular body. ( d ) Schematic of the campaniform receptor. ( e ) GFP-tubulin showing sensory cilia. ( f ) EMAP-dsRed localizes to ciliary dilations. ( g ) Merge of panels e and f (sensory cilia are marked by arrows). ( h ) Schematic of DCX-EMAP localization in chordotonal receptors. ( i ) Rhodamine-phalloidin staining the actin rods within scolopale cells. ( j ) UAS-IAV-GFP expressed in chordotonal neurons using DJ648-Gal4. ( k ) Merge showing that IAV-GFP localizes to the proximal part of the cilia. ( l ) Schematic of IAV localization. ( m ) UAS-DCX-EMAP-dsRed expressed in chordotonal neurons of Johnston's organ ( n ) UAS-CNN-GFP. ( o ) Merge of panels m and n showing the localization of DCX-EMAP-dsRed distal to CNN-GFP. ( p ) Schematic of DCX-EMAP-dsRed and CNN-GFP localization. All scale bars are 5 μm. Full size image Using DNA microarray analysis, we have determined a list of Drosophila genes in which the expression was higher in mechanoreceptor-rich tissue than in mechanoreceptor-poor tissue. Comparative qRT–PCR of RNA from the two tissues provides a partial validation of this list. Moreover, direct validation is provided by the overrepresentation of genes expressed in mechanoreceptors and genes associated with basal bodies and ciliated receptors [27] , [28] . Using this list, we identified one new candidate gene (DCX-EMAP) as the first Drosophila gene that is likely to be required for both auditory transduction and amplification, narrowing down the role of EMAP family members in the process of mechanosensation [18] and illustrating that the list contains novel molecules for mechanotransducer function. Among the candidate genes, we have shown that the microtubule-associated protein DCX-EMAP likely has a key role in Drosophila microtubule-based mechanosensation. Mechanosensation is impaired in f02655 homozygous mutants as shown by a loss of coordination and the absence of CAPs in the auditory organ. Mechanical measurements demonstrate that both mechanotransducer gating and amplification are abolished in DCX-EMAP mutants. By establishing a genetic link between mechanosensory transduction and amplification, our study corroborates theoretical studies that suggest that, at the molecular level, both processes are mechanistically linked [7] . This provides evidence that in Drosophila , not just mechanosensory transduction but also amplification is mediated by the transducer-channel complex. According to our analysis, the function of this transduction complex requires DCX-EMAP. One possibility is that DCX-EMAP is involved in intraflagellar transport (IFT), and that the flight and hearing phenotypes are due to the failure of transduction components to be correctly localized within the modified cilia. We think this is unlikely, on the basis of three arguments. First, DCX and EMAP are microtubule-associated proteins that are not known as IFT components. Second, in DCX-EMAP mutant flies, the complete cilium including dilation is present in Johnston's organ and the overall morphology of the tubular body is normal. If DCX-EMAP was an essential component of the IFT machinery, we would expect distal ciliary structures to be severely disrupted [42] . Third, we found that the inactive ion channel, which is mislocalized in IFT mutants [42] , is correctly localized in the proximal cilium of the DCX-EMAP mutant background ( Fig. 6i–l ). Thus, rather than being involved in the transport of the complex, we argue that DCX-EMAP could (1) be a part of the complex, (2) be required for proper localization of the complex, (3) participate in the coupling of mechanical forces to this complex, or (4) provide mechanical support for the complex. DCX-EMAP localizes exclusively to subcompartments of the sensory cilia, namely, the tubular body in campaniform receptors and the ciliary dilation in Johnston's organ. In DCX-EMAP mutants, these ciliary structures display specific ultrastructural defects: interfering with the DCX-EMAP function abolishes the electron-dense material between the microtubules in the tubular body and ciliary dilation while the shape of these subciliary structures is preserved. DCX-EMAP is a microtubule-binding protein and contains 10 WD domains that are known to serve as interaction platforms for other proteins [43] . We thus hypothesize that DCX-EMAP binds to microtubules within the modified sensory cilia and organizes a protein network that is visible as the electron-dense material and that may consist of diverse proteins. The defects caused by mutations in DCX-EMAP document a molecular equivalence of these materials for different types of ciliated mechanoreceptor cells. For campaniform receptors, the distal fan-shaped region of the tubular body has been hypothesized to be the site of transduction [23] . According to this hypothesis, the cuticle functions as a pair of pincers that exerts compressive force on the sensory dendrite, leading to compression of the filaments linking the dendritic sheath and plasma membrane to microtubules [6] . Our results support this hypothesis by showing that a gene, the mutation of which leads to a mechanotransduction phenotype, encodes a protein that localizes to the tubular body, and leads to ultrastructural alterations when mutated. For chordotonal receptors, the ciliary dilation has been proposed as one of the candidate sites for transduction [24] . The localization of DCX-EMAP, together with the presence of a similar electron-dense material seen in campaniform receptors, and its requirement for transduction support this idea. What role might the dilation, together with its electron-dense material, have in mechanotransduction? Because of its shape, the ciliary dilation is likely to be the weakest mechanical element along the cilium. The ciliary dilation is expected to deform when the cilium is stretched and compressed. Stretch leads to excitation of chordotonal neurons in Johnston's organ, whereas compression leads to hyperpolarization [44] . The electron-dense material may then have the role of a rigid substrate against which the channels are gated when the dilation constricts. Gating will be abolished if this mechanical support is lost, consistent with the effects seen in DCX-EMAP mutants. Our observations thus lead to a hypothesis about the mechanism of transduction channel gating in chordotonal mechanoreceptors. EMAP cloning and transgenic flies Full-length DCX-EMAP was amplified from the DGRC cDNA clone IP09257 and the short splice variant from RE01752 using the primers EMAP_fullF ATGCCACAAATTAGTCCGAACGC, CG13466F ATGTGGTATGCATCGCCTGGA, CG13466B TTCCTCGACAATGTCCCACACC and Phusion polymerase (NEB). The resulting construct was cloned into the pUAST vector [45] in frame with the coding sequence for dsRED or EYFP C terminal of the DCX-EMAP coding sequence. UAS-constructs were driven with Sca-Gal4, Elav-Gal4 or DJ648-Gal4 into campaniform receptors and chordotonal organs. Confocal microscopy was performed using a Zeiss LSM 510 Meta setup (Zeiss, Germany) or a spinning disk (IAV-GFP localization) (LEICA DMI 6000B). DNA and protein sequence analysis, as well as phylogenetic tree reconstruction, was performed using MacVector (MacVector). Stocks UAS-dsRed (Bloomington-stock number: 6282), UAS-GFP-Tubulin (7374), UAS-GFP-Cnn1 (7254), Sca-Gal4 (6479), ELAV-Gal4 (8760), DJ648-Gal4 (8172), the DCX-EMAP allele CG42247 f02655 (PBac(WH)CG42247 f02655 ), the P-element Mi(ET1)CG42247 MB00356 (22774) and deficiencies Df(3L)BSC441 (24945) and Df(3L)ED217 (8074) were obtained from the Bloomington Drosophila stock centre. Flies were raised on standard medium at 21–25 °C. The f02655 excision line was produced by precise piggyBac excision using PBac\T transposase (Flybase stock number 8285). IAV-GFP (second chromosome) stocks were kindly provided by Yun Doo Chung. Microarray probe preparation High-density oligonucleotide microarray analysis was performed using the Affymetrix Drosophila Genome1 array (Affymetrix Drosophila GeneChip microarrays, lot number 2004163 and 2004164; part number 510548; Affymetrix). Halteres of 1- to 3-day-old male and female OregonR wild-type flies were dissected and cut at the hinge between the pedicel and capitellum. Thoracic ganglion was prepared from the same flies. RNA extraction was performed using the RNeasy Mini kit (Qiagen). Amplification and labelling followed the GeneChip Eukaryotic Small Sample Target labelling assay version II (Affymetrix technical notes https://www.affymetrix.com/support/downloads/manuals/expression_s21_manual.pdf. ) Hybridization and scanning were carried out according to the standard manufacturer's protocols using the G2500A GeneArray scanner (Agilent Technologies) at 3 μm per pixel resolution at 570 nm. Arrays were scanned and quantified following the standard Affymetrix protocol. Probe level fluorescence intensities from Affymetrix CEL files were read into the R Bioconductor environment for analysis ( http://www.r-project.org , http://www.bioconductor.org ). Microarray data analysis Raw data analysis was performed using the Microarray Suite 5.0. (MAS 5.0; Affymetrix) according to Affymetrix standard procedures (Affymetrix 2002a, b). Probe sequence-dependent correction for nonspecific binding background [46] was performed using the 'affinity' model of the gcrma library: whereas 'MM' probes were used for the determination of affinity parameters, only 'PM' probes were used for probe-dependent background correction. Linear model analysis was performed using Bioconductor packages ( http://www.Bioconductor.org ) as described in detail in Supplementary Information . The latest set of annotations has been downloaded from NCBI/GEO http://www.ncbi.nlm.nih.gov/geo/ [47] . Further data analysis and data presentation were carried oute with IgorPro 5 (Wavemetrics) and Excel (Microsoft). The complete data set ( E-MEXP-1921 ) is available from ArrayExpress ( http://www.ebi.ac.uk/microarray-as/ae/ ). Flight test The flight test assay is based on Benzer [37] . Flies between 1 and 3 days of age were anaesthetized with carbon dioxide and inspected for wing defects under a stereomicroscope. Only flies without apparent wing defects were transferred to a fresh vial and allowed to recover from carbon dioxide anaesthesia for a minimum of 3 h to overnight. Usually, the number of flies per vial was 20–30. Standard 500 ml measuring cylinders were coated with paraffin oil (SIGMA, Cat. no. : 76235). Vials were opened and upturned inside a funnel. Flies falling into the cylinder initiate flight and get stuck in the paraffin oil when they hit the walls ( Fig. 2a ). The position of each fly was recorded, within 50 ml intervals of the cylinder scale. Data analysis and graphical presentation were performed with IgorPro 5 (Wavemetrics). An unpaired t -test assuming unequal variances was used for significance testing. Box plots are used for data plotting. The box marks the upper and lower quartiles (25 and 75%). Whiskers indicate the 10th and 90th percentiles. Biophysical measurements The biophysical properties of the fly's antennal sound receiver were investigated by a concurrent measurement of sound receiver mechanics and mechanically evoked nerve responses [48] . For measurements, the flies were mounted ventrum-down on top of a teflon rod with their heads, pedicels, wings, legs and halteres stabilized by wax or dental glue to minimize movements. Sound receiver mechanics were monitored at the tip of the arista using a Polytec PSV-400 Laser Doppler vibrometer (Polytec GmbH) focussed to the tip of the arista. To deduce mechanical parameters diagnostic of a ear's physiological integrity, a simple harmonic oscillator model was fitted to the power spectrum of its receiver's free fluctuations, that is, its motions in the absence of sound [49] . To measure sound-evoked responses, a receiver was stimulated with pure tones at its individual best frequency, which was determined from the free fluctuation analysis [40] . Sound stimuli were broadcast through a loudspeaker positioned ∼ 10 cm behind the fly. Stimulus intensities were monitored as the particle velocity at the receiver's position using an Emkay NR23158 pressure gradient microphone (Knowles Electronics, Itasca, IL, USA). Responses to force steps were evoked by electrostatically actuating the receiver with voltage steps fed to an electrostatic probe [7] , [38] . To this end, the experimental flies were charged to a potential value of ∼ 15 V against ground using a tungsten electrode inserted into the fly's thorax. Force-displacement characteristics were analysed by fitting a two-state gating spring model [38] to the data. Stimulus-evoked CAPs were recorded from the fly's antennal nerve by inserting an electrolytically tapered tungsten wire, serving as a different electrode, into the soft joint membrane between the first antennal segment and the head capsule [38] . The charging electrode in the fly's thorax simultaneously served as an indifferent electrode for nerve recordings. Signals were passed through a custom-built differential amplifier system and a digital noise eliminator (Hum-Bug, Quest Scientific). Electron microscopy Flies between 1 and 3 days after eclosion were anaesthetized with carbon dioxide, their halteres or Johnston's organs were dissected and these tissues were submerged in PBS containing 20% BSA (Sigma) and 0.05% pluronic acid (Sigma) [50] . Specimens were collected in cellulose capillary tubes, transferred to 100 μm-deep membrane carriers, and cryoimmobilized using an EMPACT2+RTS high-pressure freezer (Leica Microsystems) [50] . Freeze substitution was carried out in anhydrous acetone containing 1% osmium and 0.1% uranyl acetate at −90 °C up to 72 h. Samples were allowed to warm to room temperature at a rate of 5°C h −1 and thin-layer embedded in optically clean layers of Epon/Araldite on microscope slides [51] . Thin sections (70 nm) were collected on Formvar-coated copper slot grids, poststained with 2% uranyl acetate in 70% methanol, followed by Reynold's lead citrate, and imaged in a TECNAI 12 transmission electron microscope (FEI, Netherlands) operated at 100 kV. Cell culture U2OS cells stably expressing α-tubulin-mCherry [52] were grown in DME containing 10% fetal bovine serum, 2 mM l -glutamine, 100 U ml −1 penicillin, 100 μg ml −1 streptomycin and 500 μg ml −1 G418 at 37 °C in 5% carbon dioxide. Cells were transfected with full-length DCX-EMAP cloned in pCMV and tagged with C-terminal EGFP using Effectene (Qiagen) according to the supplier's protocol. How to cite this article: Bechstedt, S. et al . DCX-EMAP is a candidate gene for mechanoreception in Drosophila sensory cilia. Nat. Commun. 1:11 doi: 10.1038/ncomms1007 (2010). Copyright: © 2010 Bechstedt, S. et al . This is an open-access article distributed under the terms of the Creative Commons Attribution License, which permits unrestricted use, distribution and reproduction in any medium, provided the original author and source are credited.